Biased Brownian stepping rotation of FoF1-ATP synthase driven by proton motive force F o F 1 -ATP synthase (F o F 1 ) produces most of the ATP in cells, uniquely, by converting the proton motive force ( pmf ) into ATP production via mechanical rotation of the inner rotor complex. Technical difficulties have hampered direct investigation of pmf -driven rotation, which are crucial to elucidating the chemomechanical coupling mechanism of F o F 1 . Here we develop a novel supported membrane system for direct observation of the rotation of F o F 1 driven by pmf that was formed by photolysis of caged protons. Upon photolysis, F o F 1 initiated rotation in the opposite direction to that of the ATP-driven rotation. The step size of pmf -driven rotation was 120°, suggesting that the kinetic bottleneck is a catalytic event on F 1 with threefold symmetry. The reaction equilibrium was slightly biased to ATP synthesis like under physiological conditions, and F o F 1 showed highly stochastic behaviour, frequently making a 120° backward step. This new experimental system would be applicable to single-molecule study of other membrane proteins. F o F 1 -ATP synthase (F o F 1 ) catalyses synthesis of ATP from ADP and P i fueled by proton flux down the proton motive force ( pmf ) across biomembranes [1] , [2] , [3] . The unique feature of F o F 1 is that mechanical rotation of the inner rotor complex of F o F 1 mediates the energy conversion from pmf into ATP synthesis. F o F 1 comprises two rotary motors, F o and F 1 . F o is the transmembrane nanomotor that rotates the oligomer ring of the c -subunit against the ab 2 complex upon proton translocation. Each c -subunit has a proton-binding site and mediates proton translocation: one proton per c -subunit per rotation. Thus, the number of c -subunits in the c -ring determines the total number of protons translocated per rotation. While the number of c -subunits varies among species from 8 to 15 [4] , [5] , the bacterial F o that was used in this work has ten c -subunits to form a c 10 -ring [6] , [7] . F 1 is the protruding part of ATP synthase and an ATP-driven rotary motor that rotates the γε complex against the surrounding catalytic α 3 β 3 stator ring [8] , [9] . Each αβ interface possesses a catalytic reaction centre mainly involving the β subunits; F 1 hydrolyses three ATP molecules per turn. In a cell, the c 10 -ring and the γε complex form the common rotary shaft (red part in Fig. 1a ), while the ab 2 complex and the α 3 β 3 ring bind together via the δ subunit to form the stator complex (green part in Fig. 1a ). When pmf is sufficiently large, F o rotates the rotor complex against F 1 , leading to ATP synthesis in F 1 . When pmf diminishes, F 1 hydrolyses ATP to rotate the rotor complex in reverse, enforcing F o to pump the protons. 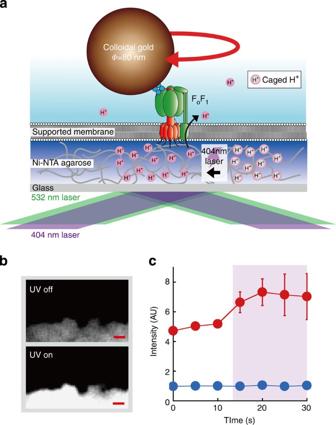Figure 1: Specifications of experimental setup. (a) Schematic model of the experimental setup. Lasers of 532 and 404 nm were introduced. The thickness of Ni-NTA agarose layer is around 200 nm. The depth of evanescent field is around 70 nm. (b) Fluorescence images of pHrodo (λex: 532 nm, λem: 575 nm) before (upper) and after (lower) ultraviolet light irradiation. The supported membrane is present in the white area. Scale bars: 2 μm. (c) Time course of the fluorescence intensity of pHrodo in the presence (red) or absence (blue) of the supported membrane. Error bars represent the s.d.’s of five measurements. The purple area represents the time period of ultraviolet light irradiation. Figure 1: Specifications of experimental setup. ( a ) Schematic model of the experimental setup. Lasers of 532 and 404 nm were introduced. The thickness of Ni-NTA agarose layer is around 200 nm. The depth of evanescent field is around 70 nm. ( b ) Fluorescence images of pHrodo (λex: 532 nm, λem: 575 nm) before (upper) and after (lower) ultraviolet light irradiation. The supported membrane is present in the white area. Scale bars: 2 μm. ( c ) Time course of the fluorescence intensity of pHrodo in the presence (red) or absence (blue) of the supported membrane. Error bars represent the s.d.’s of five measurements. The purple area represents the time period of ultraviolet light irradiation. Full size image Extensive single-molecule studies have been performed on ATP-driven rotation of F 1 to elucidate the fundamental rotation properties of F 1 , such as 120°-step rotation per turn, high unidirectionality and high coupling efficiency [10] , [11] , [12] , [13] , [14] , [15] . Most parts of the coupling reaction scheme regarding rotation and catalysis have been established, although a few uncertainties still remain [2] , [3] , [16] . On the other hand, there have been only a few studies on the rotary dynamics of F o F 1 under conditions of ATP synthesis. Single-molecule Förster resonance energy transfer (sm-FRET) has often been used to monitor the rotational dynamics of F o F 1 reconstituted in energized liposomes [17] , [18] , [19] . It was reported that F 1 makes 3-step rotations [18] , [19] while F o makes 10-step rotations, reflecting the structural symmetry of F 1 and F o (ref. 20 ). However, owing to the low signal-to-noise ratio and fast photobleaching of the dyes used in sm-FRET, high-resolution tracking of the rotational dynamics of F o F 1 has not yet been achieved. Therefore, the fundamental features of the pmf -driven rotation of F o F 1, such as the exact step size, unidirectionality of the rotation and stochasticity of the steps, remain elusive. In the present study, we attempted to directly observe the pmf -driven rotation of F o F 1 with a high spatiotemporal resolution, and revealed the fundamental features of the rotary motion of F o F 1 driven by pmf . Observation of single F o F 1 rotation driven by pmf In the present study, we have developed a novel experimental system that allows long-term recording of the single-molecule dynamics of the pmf -driven rotation of F o F 1 with a high spatiotemporal resolution. F o F 1 -reconstituted liposomes were fused to each other on a coverslip covered with Ni-NTA-modified agarose to form large supported membrane. F o F 1 molecules were anchored via His tags introduced at the periplasmic side of the oligomeric c -subunits. This connection strengthened the attachment of the lipid bilayer on the agarose sheet. The 80-nm gold colloid was attached as a rotation marker onto the β subunits of F 1 to allow visualization using the total internal reflection dark-field (TIRDF) illumination system that facilitated the long-term recording of rotation (~10 s) with a high spatiotemporal resolution of about 5 nm and<0.5 ms (ref. 21 ). In this configuration, where the rotor complex was immobilized while the stator complex rotated with the gold colloid, the pmf -driven rotation was seen to be clockwise (CW), whereas the ATP-driven rotation was counterclockwise (CCW). pmf across the supported lipid bilayer was generated by photolysis of caged proton (1-(2-nitrophenyl)ethyl sulphate) with the total internal reflection illumination of ultraviolet light light ( λ =404 nm) that selectively acidified the space between the coverslip and the lipid bilayer (the interspace). As the buffer was of high ionic strength (10 mM NaCl) compared with the generated protons, their diffusion potential (Δψ) was negligible, and thus ΔpH was essentially equal to pmf under these conditions. The magnitude of ΔpH upon photolysis of the caged protons was measured using a pH-sensitive fluorescent dye, pHrodo-Red (pHrodo) [22] , which increased the fluorescent signal upon acidification ( Supplementary Fig. S1 ). Figure 1b shows the typical time course of fluorescent response of pHrodo upon ultraviolet light irradiation. The rotation assay was conducted in the presence of 50 μM ADP, 1 μM ATP and 200 μM P i where the free energy of ATP hydrolysis, Δ G ATP , is –82 pNnm (ref. 23 ). Upon addition of nucleotides and phosphate into the flow chamber, the reconstituted F o F 1 molecules hydrolysed ATP, pumping protons from the upper open space to the interspace to generate pmf (ΔpH=+1.6±0.6) at a level of near equilibrium with Δ G ATP within a several tens of seconds ( Supplementary Fig. S2 ). Therefore, no rotating particles were observed before ultraviolet light irradiation; the average rate was 0 r.p.s. before ultraviolet light irradiation ( Fig. 2b ), implying non-biased rotary Brownian motion. Upon the ultraviolet light irradiation, some particle showed continuous rotation. We arbitrarily selected particles showing rotational fluctuation before ultraviolet light irradiation and observed after uncaging for 5–31 s. About 11.5% of the observed particles (38/330 particles) showed continuous rotation in CW direction over five turns within the observation time as expected ( Fig. 2a ). The averaged velocity was 2.7 r.p.s. Although most of the particles terminated the rotation abruptly, probably because of ultraviolet light-inactivation or nonspecific attachment to the substrate in most cases, some molecules still retained the activity after ultraviolet light irradiation, which was confirmed by ATP-driven CCW rotation after injection of an ATP solution ( Supplementary Fig. S3 ). For further confirmation of the rotation driven by pmf , we tested the effect of a specific inhibitor of F o , N , N ′-dicyclohexylcarbodiimide (DCCD) [24] , on the rotation. When F o F 1 was treated with 200 μM DCCD, none of particles showed rotation (0/273 particles), supporting the validity of the experiment. The pmf -driven rotation was also observed in the absence of ADP and P i ( Fig. 2c ). The average velocity was 6.6 r.p.s., faster than that in the presence of nucleotides ( Fig. 2d ). This is probably because the nucleotide-depleted F 1 has a threefold rotary potential with lower energy barriers compared with ATP-synthesizing F 1 as discussed below. Another line of our experiment also suggested that energetic barrier of the rotary potential of nucleotide-depleted F 1 is low; around 4–5 k B T (Fujisawa et al ., unpublished data). 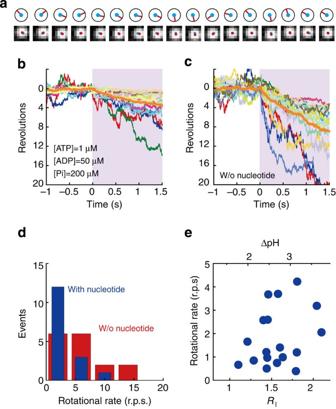Figure 2: Rotary motion of FoF1in the presence of ΔpH. (a) Sequential images of a rotating particle in the presence of ΔpH (lower). Blue and red points represent the centre of the rotation and the centroid of the gold nanoparticle, respectively. The angular positions of the particle are shown in the upper figures. The interval between images is 5 ms. Time course of the rotation of FoF1in the presence (b) or absence (c) of nucleotides. The purple area (t>0 s) represents the time period of ultraviolet light irradiation. The solid orange lines represent the averaged time course from 17–18 molecules. (d) Histogram of the rotational speed in the absence (red) or presence (blue) of nucleotides. (e) Rotational speed plotted against the relative increment of the fluorescence of pHrodo,RI(or ΔpH, seeSupplementary Fig. S1). Figure 2: Rotary motion of F o F 1 in the presence of ΔpH. ( a ) Sequential images of a rotating particle in the presence of ΔpH (lower). Blue and red points represent the centre of the rotation and the centroid of the gold nanoparticle, respectively. The angular positions of the particle are shown in the upper figures. The interval between images is 5 ms. Time course of the rotation of F o F 1 in the presence ( b ) or absence ( c ) of nucleotides. The purple area ( t >0 s) represents the time period of ultraviolet light irradiation. The solid orange lines represent the averaged time course from 17–18 molecules. ( d ) Histogram of the rotational speed in the absence (red) or presence (blue) of nucleotides. ( e ) Rotational speed plotted against the relative increment of the fluorescence of pHrodo, R I (or ΔpH, see Supplementary Fig. S1 ). Full size image ΔpH dependence of the rotational rate To investigate the correlation between the rotational rate and ΔpH, the fluorescent response of pHrodo was measured in the region where F o F 1 showed rotations under conditions of ATP synthesis ( Supplementary Fig. S4 ). As pHrodo readily photobleaches under co-illumination of ultraviolet light and 532 nm excitation, the simultaneous imaging of TIRDF and fluorescent imaging of pHrodo was not possible. As an alternative, ΔpH formed upon ultraviolet light irradiation was estimated as follows. Ultraviolet light laser was switched off to terminate the observation of pmf -driven rotation. After 5 min elapsed and pHrodo recovered the original fluorescence intensity before ultraviolet light irradiation, ultraviolet light laser was again irradiated on specimen and the fluorescence image of pHrodo around the rotating particle (2.5 × 2.5 μm 2 ) was recorded with intermittent illumination of 532 nm for 240 ms with 5 s intervals. The relative increment of the fluorescence upon ultraviolet light irradiation ( R I ) was plotted against the averaged velocity of rotating particles ( Fig. 2e ). ΔpH was determined from R I taking into account that ΔpH of +1.6 was created by the proton-pumping activity of F o F 1 before ultraviolet light irradiation. Although F o F 1 showed a large variation in velocity, it is still evident that faster rotation occurred at high ΔpH. It is likely that the slow rotation at high ΔpH was caused by physical hindrance or nonspecific interaction with the lipid bilayer. The data points of higher velocity at a given ΔpH qualitatively agreed with the previous biochemical measurement [25] , supporting the validity of our measurement. Stepping rotation Stepping behaviour of the rotating particle before and after ultraviolet light irradiation was analysed. The rotating particle demonstrated remarkably large rotary fluctuation during pmf -driven rotation. This is a prominent feature of the pmf -driven rotation of F o F 1 that is not seen in the ATP-driven rotation of F 1 or F o F 1 . Some molecules showed clear 120° forward-and-backward steps (insets of Fig. 3a ). This 120° stepping was also observed in the absence of pmf ( Fig. 3b ), suggesting that pmf biased the rotary diffusion to the CW direction. Although rotation without nucleotides also showed 3-step rotation, the 120° steps were obscure ( Supplementary Fig. S5 ). From the analysis of the histograms of angular positions, the rotary potentials of F o F 1 were determined according to Boltzmann’s Law ( Supplementary Fig. S6 ). The rotary potential without nucleotide was much more gradual than that with nucleotide, suggesting that the first-passage time to overcome the potential barrier should become longer in the presence of nucleotides, that is, the rotational speed becomes slower, which is consistent with the aforementioned experimental result ( Fig. 2d ). Hereafter, rotation was only analysed in the presence of nucleotides. 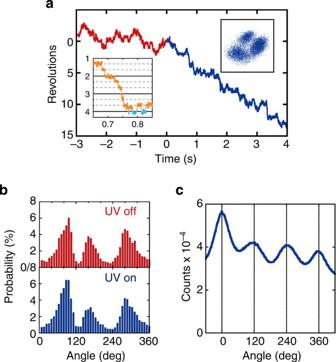Figure 3: Stepping rotation of FoF1. (a) Time course of the stepping rotation of FoF1in the presence of 50 μM ADP, 1 μM ATP and 200 μM Pibefore (red) and after (blue) ultraviolet light irradiation. The left inset presents an enlarged view of the time course. Orange and light blue points represent the pauses before CW and CCW steps, respectively. The right inset is the centroid trajectory of the rotating particle during ultraviolet light irradiation. (b) Histograms of the angular positions before (upper) or after (lower) ultraviolet light irradiation in the presence of 50 μM ADP, 1 μM ATP and 200 μM Pi. (c) Histogram of the pairwise distribution of the angular displacement derived from the time courses of the rotation in the presence of 50 μM ADP, 1 μM ATP and 200 μM Pi. The histogram is derived from 42 rotations of three molecules. The window size of the analysis is Δt=0.5–1,000 ms. Figure 3: Stepping rotation of F o F 1. ( a ) Time course of the stepping rotation of F o F 1 in the presence of 50 μM ADP, 1 μM ATP and 200 μM P i before (red) and after (blue) ultraviolet light irradiation. The left inset presents an enlarged view of the time course. Orange and light blue points represent the pauses before CW and CCW steps, respectively. The right inset is the centroid trajectory of the rotating particle during ultraviolet light irradiation. ( b ) Histograms of the angular positions before (upper) or after (lower) ultraviolet light irradiation in the presence of 50 μM ADP, 1 μM ATP and 200 μM P i . ( c ) Histogram of the pairwise distribution of the angular displacement derived from the time courses of the rotation in the presence of 50 μM ADP, 1 μM ATP and 200 μM P i . The histogram is derived from 42 rotations of three molecules. The window size of the analysis is Δ t =0.5–1,000 ms. Full size image Pairwise distance analysis of the rotation of six molecules also showed evident peaks with 120° intervals ( Fig. 3c ). We also explored the possibility of 36° steps caused by the rotary potential minima of F o that has tenfold symmetry [6] . However, no signs of 36° steps were found in angle histograms of pairwise analysis. This implies that the rotary potential of F 1 with threefold symmetry dominated the overall rotary potential of the rotor shaft in F o F 1 . In other words, the kinetic bottleneck of the pmf -driven rotation in the present condition is not proton translocation in F o but a catalytic event(s) on F 1 -ATPase, such as ATP release or P i binding, as previous studies suggested [26] , [27] . For the molecules with clear, discrete 120° steps, the pause durations between the 120° steps were analysed ( Fig. 3a , inset). Before ultraviolet light irradiation, the histograms of the pause duration before CW or CCW rotation were essentially identical, showing single exponential decay ( Fig. 4a ). The rate constants of the CW and CCW steps ( k cw and k ccw ) were determined to be 65 and 61 s −1 , respectively ( Fig. 4a ). The equilibrium constant of CW rotation ( K E CW ) was, thus, almost 1. Under ultraviolet light irradiation, k cw markedly increased to 100 s −1 , while k ccw slightly decreased to 48 s −1 ( Fig. 4b ). Resultantly, K E CW under ultraviolet light irradiation increased to 2 ( Fig. 4c ), implying that pmf biased step direction. 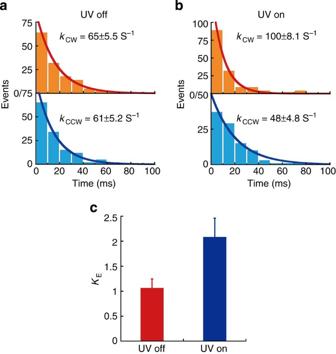Figure 4: Kinetic analysis of the rotary motion of FoF1. Histograms of the pause durations before (a) or after (b) ultraviolet light irradiation in the presence of 50 μM ADP, 1 μM ATP and 200 μM Pi. The upper and lower figures represent the histograms before CW and CCW steps, respectively. Solid lines represent the fitted curve based on the single exponential decay functions. Each histogram is composed of 99–152 durations from three molecules. Error is given as, whereNis the number of durations. (c) Equilibrium constants (KECW=kcw/kccw) determined from (a) or (b). Error bars represent the errors of the equilibrium constants propagated from those in (a) or (b). Figure 4: Kinetic analysis of the rotary motion of F o F 1. Histograms of the pause durations before ( a ) or after ( b ) ultraviolet light irradiation in the presence of 50 μM ADP, 1 μM ATP and 200 μM P i . The upper and lower figures represent the histograms before CW and CCW steps, respectively. Solid lines represent the fitted curve based on the single exponential decay functions. Each histogram is composed of 99–152 durations from three molecules. Error is given as , where N is the number of durations. ( c ) Equilibrium constants ( K E CW = k cw / k ccw ) determined from ( a ) or ( b ). Error bars represent the errors of the equilibrium constants propagated from those in ( a ) or ( b ). Full size image This study verified that F o F 1 rotates CW, by directly observing the rotation of F o F 1 in the presence of pmf The step size of the rotation was 120°. The 36° substeps reflecting the structural symmetry of F o were not observed. This implies that the rate-determining step is a catalytic event of F 1 . This result is consistent with a previous sm-FRET measurement of rotation of F o F 1 in ATP synthesis condition where a pair of FRET probes were introduced at a stator of F o and a rotor subunit of F 1 (refs 18 , 19 ), while small steps that was estimated to be 36° were recorded when FRET probes were introduced into F o (ref. 17 ). In the present study, we immobilized the rotor part of F o on a coverslip and attached the rotation probe at the stator part of F 1 . Therefore, the observed rotation reflects the stepping behaviour both of F 1 and F o as shown in the other works, in which 36° steps of ATP-driven rotation of F o F 1 were observed in a similar experimental setup [20] . However, we do not exclude the possibility that the difference in the probe position caused the apparently different step size of the rotation. Another possible reason why 36° substeps were not found is that the elasticity of the rotor complex makes 36° substeps in 120° step obscure [28] , [29] . In addition, the difference in the components of pmf could also explain the inconsistency in step size; while pmf in the sm-FRET measurements was composed both of ΔpH and Δψ, pmf was essentially composed only of ΔpH in the present study. The stochastic CW and CCW 120° stepping rotation was another new finding of the present study. As pmf did not fully dominate the free energy of ATP hydrolysis, the chemical equilibrium was slightly biased towards ATP synthesis and F o F 1 made frequent backward steps of 120°. Although the nucleotide concentrations are different from those under intracellular conditions, the stochastic rotation would represent rotation under physiological conditions where the torque of F o almost balances that of F 1 . A similar stochastic 120° stepping rotation has been reported for the rotation of isolated F 1 under opposing torque that mimics the torque of F o (ref. 12 ). This work also presented a new experimental strategy for the single-molecule investigations of membrane proteins of which the driving force is the electrochemical potential. Although various kinds of artificial membrane systems have been studied in the past, it has been remarkably difficult to observe the conformational dynamics of membrane proteins driven by electrochemical potential at the single-molecule level. As there are several caged compounds that release specific ions or chemicals, the present approach can also be applied to single-molecule studies of transporters and ion channels. Protein preparations and reconstitution into liposome The mutant F o F 1 from E. coli , which lacks the two α-helices in the C-terminus of the ε subunit and has a His 3 -tag and a biotin-binding domain in the c and β subunit, respectively, and KcsA were expressed, purified and reconstituted to the liposome, as previously reported with slight modification [25] , [30] . In short, liposome was prepared from the 1:1 (w:w) mixture of 1,2-dioleoyl- sn -glycero-3-phosphoethanolamine (NOF Cooperation) and 1,2-dioleoyl- sn -glycero-3-phosphoglycerol (DOPG, NOF cooperation) by reverse-phase evaporation. To reconstitute F o F 1 and KcsA to the same liposome, we mixed these proteins to a final concentration of ~0.07 mg/ L for F o F 1 and 0.04 mg/ L for KcsA. The mixture was sonicated for 10 s at room temperature. To suppress ion leakage, a potassium channel protein, KcsA, which confers greater sealing to lipid bilayers ( Supplementary Fig. S7 ), was co-reconstituted with F o F 1 . Although the mechanism of this phenomenon is unknown, the effect of KcsA reconstitution to suppress proton leakage was confirmed in our experimental setup ( Supplementary Fig. S8 ). Potassium ions were not included in the buffer to avoid possible potassium leakage. Ni-NTA agarose glass preparation The Ni-NTA agarose glass was prepared in three steps. The first step entailed the preparation of glycidol–agarose gel. We extensively washed 20 ml of agarose beads (Sepharose 4B, Sigma) with distilled water, and they were suspended in 180 ml of distilled water. Then, 100 ml of a solution containing 1 M NaOH, 26 mM NaBH 4 and 20 ml of glycidol was added, and the reaction mixture was incubated at room temperature for 18 h. The product was alternatively washed with distilled water and 1 M NaCl, and the glycidol–agarose beads were prepared. The second step involved the preparation of aldehyde-activated agarose beads by periodate oxidation of the glycidol–agarose beads. The glycidol–agarose beads were diluted in 250 ml of distilled water. Then, 70 ml of 0.16 M NaIO 4 was added, and the mixture was incubated at room temperature for 1 h. The product was extensively washed with distilled water, yielding the aldehyde-activated agarose beads. The last step involved the agarose coating of the glass surface and the coupling of AB-NTA (Dojindo) to prepare the Ni-NTA agarose glass. The aldehyde-activated agarose beads were diluted in distilled water, and boiled at 100 °C for 10 min. The melted aldehyde-activated agarose was spin-coated onto the coverslip at 3,000 r.p.s. for 20 s. After coating, the glass was immersed in 1 M boric acid-NaOH buffer (pH 10.5) containing 26 mg ml −1 of AB-NTA and 12 mg ml −1 of NaCNBH 3 for 16 h at room temperature. The NTA agarose glass was washed with distilled water and immersed for 1 day in an aqueous solution containing 1 mM NiSO 4 . Microscopy We observed the gold nanoparticles ( φ = 80 nm) with the TIRDF illumination system equipped on an Olympus IX-71 microscope [21] . The evanescent fields of two kinds of laser light (wavelength: 532 and 404 nm) were formed on the Ni-NTA agarose glass for illuminating the gold nanoparticles (532 nm), exciting pHrodo-Red (532 nm) and uncaging the caged proton (404 nm). The laser powers at the base of the objective ( × 60; NA1.49; Olympus) were 3.3 mW for 532 nm, and 0.1 mW for 404 nm, which illuminated 1,800 μm 2 at the sample plane. The fluorescence (pHrodo-Red) and dark-field (gold nanoparticle) images were separated with a dichroic mirror and recorded with two cameras: Electron Multiplying CCD; EMCCD (iXon, Andor) and fast-frame CMOS camera (FASTCAM-1024PCI, Photron). Supported membrane formation and rotation assay of F o F 1 In order to visualize the rotary motion of F o F 1 , we immobilized the stator part (red part in Fig. 1a ) on the glass surface and attached the gold nanoparticle to the rotor part (green part in Fig. 1a ) to probe the rotation. We prepared the sample as follows. At first, the liposomes, in which F o F 1 and KcsA were reconstituted, were spotted onto the surface of Ni-NTA agarose glass and dried in air for 10 min. Before spotting, glycerol (1% in final) was added in the sample to avoid complete desiccation. Then, to form the supported bilayer membrane, we dropped buffer A (10 μM MOPS-KOH (pH 8.0), 10 mM NaCl, 10 mM 1-(2-nitrophenyl)ethyl sulphate (NPE-caged proton, Tocris Bioscience), which contained an indicated amount of substrates, that is, Mg-ADP, Mg-ATP and P i , onto the liposome spot. After 2 h had elapsed, we placed two spacers of 50 μm-thickness and a coverslip onto the plate to create a flow cell. A mixture of the gold nanoparticle ( φ = 80 nm, prepared as described previously [21] ) and substrates in buffer A was infused into the flow cell, and commenced observation of the rotary motion of F o F 1 by introducing the evanescent waves of 532 and 404 nm lasers. Some gold nanoparticles, which were attached to F o F 1 , showed the two-dimensional diffusion, and therefore, the liposomes were found to be converted into a planar membrane during aforementioned process. The rotating gold nanoparticles were recorded as an eight-bit AVI file with a fast-frame camera (1024 PCI, Photron) at 2,000 fps. For photolysis of caged proton, we used illumination by the evanescent waves of 404 nm. The rotation assay was performed at 23 °C. Fluorescence imaging of pHrodo-Red In order to measure the amplitude of pH, we infused buffer A containing 3 μM pHrodo-Red (Invitrogen), into the flow cell. The fluorescence image of pHrodo-Red was recorded by EMCCD camera (iXon, Andor) at 16.7 f.p.s. ΔpH measurement We measured the magnitude of ΔpH across the membrane generated upon photolysis of caged protons using the pH-sensitive fluorescent dye, pHrodo-Red, that increased the fluorescent signal upon acidification ( Fig. 1b ). Although pHrodo-Red was preferentially localized on the bilayer surface, it responded well to acidification of the space between the bilayer and the coverslip, showing the same tendency as that obtained in a control bulk experiment ( Supplementary Fig. S1 ). The pH of the interspace was determined from the fluorescent signal change ( R I ), taking into account that only the dyes located under the supported membrane increase fluorescence intensity upon ultraviolet light irradiation. Although caged protons above the bilayer were somehow uncaged, it did not affect the net fluorescence intensity, because the upper solution was virtually opened upward so that the released protons immediately diffused outward. For the proton-pump activity measurement of F o F 1 driven by ATP hydrolysis, caged-ATP (Dojindo) was used. How to cite this article: Watanabe, R. et al . Biased Brownian stepping rotation of F o F 1 -ATP synthase driven by proton motive force. Nat. Commun. 4:1631 doi: 10.1038/ncomms2631 (2013).